A monomeric red fluorescent protein with low cytotoxicity Multicolour labelling with fluorescent proteins is frequently used to differentially highlight specific structures in living systems. Labelling with fusion proteins is particularly demanding and is still problematic with the currently available palette of fluorescent proteins that emit in the red range due to unsuitable subcellular localization, protein-induced toxicity and low levels of labelling efficiency. Here we report a new monomeric red fluorescent protein, called FusionRed, which demonstrates both high efficiency in fusions and low toxicity in living cells and tissues. The majority of applications for fluorescent protein fusions strictly require a monomeric state to minimize artifacts that often occur when fusion proteins are expressed at concentrations that exceed those of the endogenous protein. Many fusion constructs, and most fluorescent protein-based biosensors, are critically sensitive to oligomerization, non-specific subcellular localization or secondary protein–protein interactions, as well as possible aggregation. It was fortuitous that the first fluorescent protein to be successfully cloned, Aequorea victoria green fluorescent protein (GFP), was naturally monomeric at intracellular expression levels and thus suitable for protein labelling in living cells. Unfortunately, the majority of green and yellow and all of the red-emitting fluorescent proteins derived from non- Aequorea species are dimeric or tetrameric in nature. This undesirable oligomerization feature was a sticking point for many years until Tsien et al . [1] designed, in 2002, the first monomeric red fluorescent protein, mRFP1, which was derived from naturally tetrameric DsRed [2] . Over the past decade, a number of red dimeric and tetrameric fluorescent proteins have been subjected to artificial monomerization, which in most cases has resulted in a loss of brightness, a slower maturation rate and reduced fluorescence stability. Engineered red monomers, such as mCherry and other mFruit proteins [3] , along with mKO [4] , TagRFP [5] and mKate2 (refs 6 , 7 ) are suitable fusion partners for many proteins of interest. However, these proteins usually do not perform as well as Aequorea victoria GFP derivatives in fusions, and often present issues related to abnormal subcellular protein localization, aggregation, or toxic effects [8] . Such behaviour is most likely due to a residual tendency of non- Aequorea fluorescent proteins to dimerize or as the result of unpredictable interactions between newly exposed and modified hydrophobic surfaces of engineered monomeric variants. In this work, we report a low toxicity monomeric red fluorescent protein, named FusionRed, which exhibits a high level of performance in fusions, comparable to that of the best green fluorescent protein variants. Development of a purely monomeric red fluorescent protein The previously reported bright, far-red fluorescent protein mKate2 appeared to be the best variant to start with due to its proven performance in the majority of fusion constructs, low toxicity in Xenopus laevis embryos, and absence of visible aggregates or non-specific localization in mammalian cells at high expression levels. With low-pressure liquid chromatography, we earlier demonstrated that mKate2 is monomeric in character at concentrations (loaded onto a column) of up to 10 mg ml −1 (ref. 7 ). However, high-pressure liquid chromatography (HPLC) reveals the presence of an equilibrium monomer–dimer fraction of mKate2 ( Fig. 1 and ref. 9 ), which is most probably due to the higher protein concentrations achieved in the absence of significant dilution during chromatography. We believe that this residual dimerization tendency could potentially affect the optimal performance of mKate2 in certain fusions. Here, we aimed to develop a purely monomeric (at high concentrations as verified by HPLC) version of mKate2 that would inherit its low toxicity and its nominal tendency to aggregate in living cells. 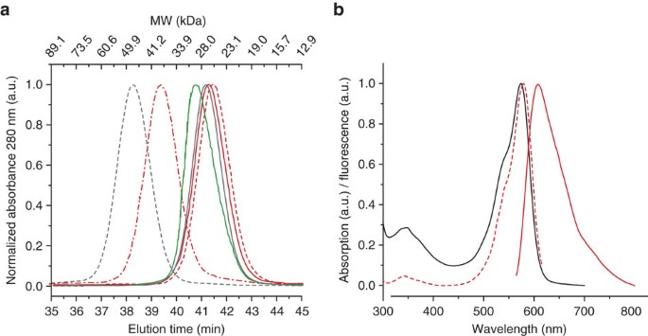Figure 1: In vitro characterization of FusionRed. (a) HPLC results for FusionRed (solid red line), mKate2.5 (dashed red line), mKate2 (dot-dashed red line), mCherry (solid grey line), mEGFP (solid green line) and mNeptune (dotted grey line). Proteins were loaded at a concentration of 10 mg ml−1. (b) FusionRed absorption (solid black line), excitation (dashed red line) and emission (solid red line) spectra. Figure 1: In vitro characterization of FusionRed. ( a ) HPLC results for FusionRed (solid red line), mKate2.5 (dashed red line), mKate2 (dot-dashed red line), mCherry (solid grey line), mEGFP (solid green line) and mNeptune (dotted grey line). Proteins were loaded at a concentration of 10 mg ml −1 . ( b ) FusionRed absorption (solid black line), excitation (dashed red line) and emission (solid red line) spectra. Full size image Our strategy involved analyzing recently obtained crystallographic data of the structure of mKate [10] (PDB ID: 3BXB) and choosing a set of amino-acid residues that would affect oligomerization for further site-directed mutagenesis. In addition, we substituted the hydrophobic C-terminal tail that stabilizes mKate dimers ( Fig. 2 )—which might possibly alter its performance in fusion constructs—with a flexible Gly-rich linker. In total, the following mutations: S132A, R164A, K182E, Y200N were inserted and, along with the substituted C-terminus, yielded a variant named mKate2.5 (see Supplementary Fig. S1 for alignment), characterized by monomeric behaviour at 10 mg ml −1 concentrations on HPLC ( Fig. 1a ). 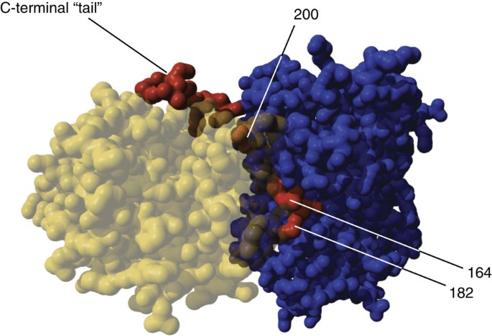Figure 2: Visualization of the amino-acid positions responsible for mKate dimerization. The Figure depicts a structural model based on mKate crystallographic data10. Amino-acid residues responsible for dimerization are shown in orange and numbers in the sequence are stated. The two mKate subunits are coloured yellow (semitransparent) and blue. Figure 2: Visualization of the amino-acid positions responsible for mKate dimerization. The Figure depicts a structural model based on mKate crystallographic data [10] . Amino-acid residues responsible for dimerization are shown in orange and numbers in the sequence are stated. The two mKate subunits are coloured yellow (semitransparent) and blue. Full size image Maturation rate, fluorescence brightness and pH stability of mKate2.5 were significantly reduced compared with mKate2 (data not shown). To rescue the protein’s spectral and biochemical properties, several rounds of combined site-directed and random mutagenesis were performed. After each round of random mutagenesis, all variants containing substitutions that would likely lead to oligomerization were ignored, whereas potentially beneficial mutations were combined in the next rounds of mutagenesis. A number of substitutions were introduced during the random mutagenesis, including a duplet of proline residues (T75P, Q76P) between the chromophore-carrying α-chain and the fourth β-strand, which produced the most significant positive effect on protein maturation. These substitutions indicated that the disturbed β-barrel of the monomeric protein required significant twist in this loop. The mutations K69R and R203H in the region surrounding the chromophore from a close homologue, TagRFP ( Supplementary Fig. S1 ), were transferred to mKate2.5 and resulted in dramatically enhanced pH stability of the protein along with a 25-nm hypsochromic shift of the emission maximum ( Fig. 1b ). The final variant, named FusionRed, demonstrates brightness comparable to that of mKate2 ( Table 1 ). Other important characteristics (including pH stability, photostability and maturation rate) are also comparable to current red-emitting fusions of practical value ( Table 1 ). Table 1 Key characteristics of selected monomeric red fluorescent proteins. Full size table Although HPLC demonstrates reversible dimerization of mKate2 and reveals a dimeric character for the mKate derivative, far-red fluorescent protein mNeptune [9] , FusionRed—along with monomeric Enhanced GFP (mEGFP) (considered to be the ‘gold standard’)—behaves as a pure monomer at concentrations up to 10 mg ml −1 ( Fig. 1a ). It should be noted that the popular red fluorescent protein, mCherry [3] , also behaves as a pure monomer with HPLC analysis ( Fig. 1a ), but its performance as a reporter in fusion constructs is not always satisfactory [8] . Thus, monomeric character seems to be necessary but not sufficient for optimal performance in fusions. Performance of FusionRed in fusions To test FusionRed performance in fusions, we have generated chimeric constructs with more than 40 proteins of interest ( Fig. 3 and Supplementary movies 1 , 2 , 3 , 4 , 5 , 6 , 7 , 8 ). Owing to the lack of a statistical methodology to make direct comparisons of fluorescent protein performance in fusions, the practice is utilized only to provide one or several representative images that demonstrate the ability of the reporter to properly perform in each of the constructs. However, as it has been noted [8] , the expression level range that provides for acceptable performance is much narrower for red monomers when compared with the best green fluorescent proteins. Therefore, it was critical that FusionRed consistently performed well at both low and high expression levels, which are always produced during transient transfections. Our subjective impression was that the performance of FusionRed is comparable to that of the best green fluorescent proteins, such as mEGFP or mEmerald, and is one of the best compared to other available red fluorescent proteins. 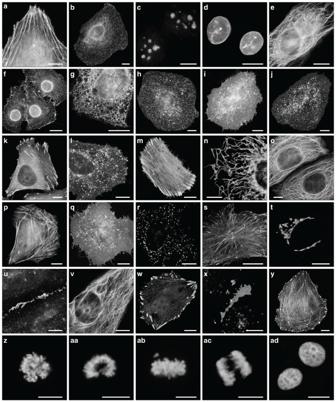Figure 3: Fluorescence imaging of FusionRed fusion vectors. (a–l) C-terminal FusionRed fusion constructs; for each fusion protein the linker amino-acid length is indicated after the name of the targeted organelle or fusion protein: (a) FusionRed-β-actin-18 (human); (b) FusionRed-Rab5a-7 (canine; endosomes); (c) FusionRed-fibrillarin-7 (human; nucleoli); (d) FusionRed-lamin B1-10 (human); (e) FusionRed-α-tubulin-18 (human); (f) FusionRed-annexin (A4)-12 (human); (g) FusionRed-endoplasmic reticulin-5 (calreticulin signal and KDEL; human); (h) FusionRed-caveolin1-10 (human); (i) FusionRed-CAAX-5 (20-amino-acid farnesylation signal from c-Ha-Ras; membrane); (j) FusionRed-endosomes-14 (human RhoB GTPase and c-Myc epitope tag). (k–y) N-terminal fusion constructs; (k) FusionRed-Paxillin-22 (chicken); (l) FusionRed-LAMP1-20 (rat; lysosomal membrane glycoprotein 1); (m) FusionRed-Lifeact-7 (yeast; actin); (n) FusionRed-PDHA1-10 (human; pyruvate dehydrogenase; mitochondria); (o) FusionRed-keratin-17 (human; intermediate filaments; cytokeratin 18); (p) FusionRed-light chain myosin-7 (mouse); (q) FusionRed-c-src-N-7 (chicken); (r) FusionRed-PMP-10 (human peroxisomal membrane protein); (s) FusionRed-EB3-7 (human microtubule-associated protein; RP/EB family); (t) FusionRed-SiT-15 (N-terminal 45 amino acids of human sialyltransferase; Golgi); (u) FusionRed-VE-Cadherin-10 (human); (v) FusionRed-vimentin-7 (human); (w) FusionRed-zyxin-7 (human); (x) FusionRed-Cx43-7 (rat α-1 connexin-43); (y) FusionRed-α-actinin-19 (human; non-muscle). (z–ad) FusionRed-H2B-C-10 (human) in HeLa S3 cells; (z) prophase; (aa) prometaphase; (ab) metaphase; (ac) anaphase; (ad) interphase. The cell line used for expression FusionRed constructs was human cervical adenocarcinoma cells (HeLa; ATCC, S3) ind,f,oandz–ad. African green monkey kidney cells (ATCC, CV-1) were used ins, and HeLa CCL2 (ATCC) cells were used in the remaining panels. Scale bars represent 10 μm. Figure 3: Fluorescence imaging of FusionRed fusion vectors. ( a – l ) C-terminal FusionRed fusion constructs; for each fusion protein the linker amino-acid length is indicated after the name of the targeted organelle or fusion protein: ( a ) FusionRed-β-actin-18 (human); ( b ) FusionRed-Rab5a-7 (canine; endosomes); ( c ) FusionRed-fibrillarin-7 (human; nucleoli); ( d ) FusionRed-lamin B1-10 (human); ( e ) FusionRed-α-tubulin-18 (human); ( f ) FusionRed-annexin (A4)-12 (human); ( g ) FusionRed-endoplasmic reticulin-5 (calreticulin signal and KDEL; human); ( h ) FusionRed-caveolin1-10 (human); ( i ) FusionRed-CAAX-5 (20-amino-acid farnesylation signal from c-Ha-Ras; membrane); ( j ) FusionRed-endosomes-14 (human RhoB GTPase and c-Myc epitope tag). ( k – y ) N-terminal fusion constructs; ( k ) FusionRed-Paxillin-22 (chicken); ( l ) FusionRed-LAMP1-20 (rat; lysosomal membrane glycoprotein 1); ( m ) FusionRed-Lifeact-7 (yeast; actin); ( n ) FusionRed-PDHA1-10 (human; pyruvate dehydrogenase; mitochondria); ( o ) FusionRed-keratin-17 (human; intermediate filaments; cytokeratin 18); ( p ) FusionRed-light chain myosin-7 (mouse); ( q ) FusionRed-c-src-N-7 (chicken); ( r ) FusionRed-PMP-10 (human peroxisomal membrane protein); ( s ) FusionRed-EB3-7 (human microtubule-associated protein; RP/EB family); ( t ) FusionRed-SiT-15 (N-terminal 45 amino acids of human sialyltransferase; Golgi); ( u ) FusionRed-VE-Cadherin-10 (human); ( v ) FusionRed-vimentin-7 (human); ( w ) FusionRed-zyxin-7 (human); ( x ) FusionRed-Cx43-7 (rat α-1 connexin-43); ( y ) FusionRed-α-actinin-19 (human; non-muscle). ( z – ad ) FusionRed-H2B-C-10 (human) in HeLa S3 cells; ( z ) prophase; ( aa ) prometaphase; ( ab ) metaphase; ( ac ) anaphase; ( ad ) interphase. The cell line used for expression FusionRed constructs was human cervical adenocarcinoma cells (HeLa; ATCC, S3) in d , f , o and z – ad . African green monkey kidney cells (ATCC, CV-1) were used in s , and HeLa CCL2 (ATCC) cells were used in the remaining panels. Scale bars represent 10 μm. Full size image To further illustrate the capability of FusionRed as a red-emitting reporter, we directly compared the performance of FusionRed and mCherry in HeLa CCL2 cells for the following targets: connexin-43, endosomes, vinculin and the Golgi complex. In this experiment, HeLa CCL2 cells were transfected with each of the four target fusions, fixed and then compared for localization efficiency, which was determined by calculating the percentage of properly expressing cells versus the total number of transfected cells. FusionRed consistently outperformed mCherry in the four fusions with 76, 63, 58 and 42% of the transfected population of cells properly localizing connexin-43, endosomes, vinculin and Golgi, respectively. Properly localizing cell populations of mCherry fusions of connexin-43, endosomes, vinculin and Golgi, however, only constituted 28, 21, 37 and 30% of transfected cells, respectively ( Supplementary Fig. S4 ). FusionRed cytotoxicity Another important characteristic we considered in the development of this new reporter, especially for long-term imaging, was protein cytotoxicity in living cells. To do so, we evaluated cytotoxicity of selected red fluorescent proteins relative to EGFP in the following experiment: HeLa cells were transfected with appropriate vectors encoding EGFP or one of the following red fluorescent proteins: mRuby [11] , FusionRed, mKate2 or mCherry. Next, the EGFP-expressing cells were mixed with those expressing one of the RFPs, resulting in four separate cell mixtures: EGFP and mRuby, EGFP and FusionRed, EGFP and mKate2, and EGFP and mCherry. Forty-eight hours after transfection, the green-to-red cell ratios were calculated utilizing flow cytometry and each of the cell mixtures were then plated into three plates. After additional 92 h incubation, the green-to-red cell ratios were recalculated. Because only living cells were counted for this experiment, the difference between the ratios before and after the incubation can be assumed to accurately reflect RFP toxicity versus EGFP. mRuby exhibited a more than 10-fold higher cytotoxicity level compared with EGFP, whereas the remaining RFPs were almost as cytotoxic as EGFP in this experiment ( Fig. 4 ). 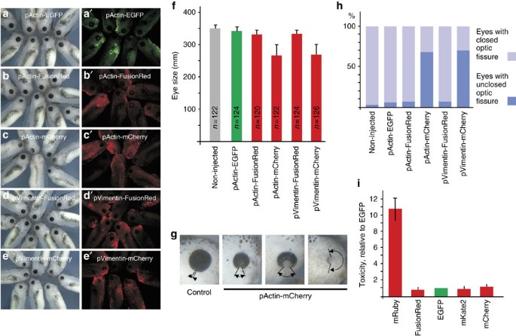Figure 4: In vivo toxicity of selected fluorescent proteins. (a–e′) Stage 41Xenopus laevistadpoles expressing fluorescent protein fusions. (a-e) White light; (a′–e′) fluorescence. (f) Mean values of eye size ofXenopus laevisembryos injected with plasmids expressing different fluorescent protein fusions. (g) Examples of the tadpole eyes injected by pActin-mCherry plasmid demonstrate different degrees of optic fissure closure. The control eye is of the non-injected tadpole. Arcs ending by arrowheads indicate radial angles formed by the edges of unclosed optic fissures. Dorsal to the top, anterior to the right. (h) Score of eyes with closed and unclosed optic fissure. (i) Protein cytotoxicity in HeLa cells relative to EGFP. Figure 4: In vivo toxicity of selected fluorescent proteins. ( a – e′ ) Stage 41 Xenopus laevis tadpoles expressing fluorescent protein fusions. ( a-e ) White light; ( a′ – e′ ) fluorescence. ( f ) Mean values of eye size of Xenopus laevis embryos injected with plasmids expressing different fluorescent protein fusions. ( g ) Examples of the tadpole eyes injected by pActin-mCherry plasmid demonstrate different degrees of optic fissure closure. The control eye is of the non-injected tadpole. Arcs ending by arrowheads indicate radial angles formed by the edges of unclosed optic fissures. Dorsal to the top, anterior to the right. ( h ) Score of eyes with closed and unclosed optic fissure. ( i ) Protein cytotoxicity in HeLa cells relative to EGFP. Full size image Notably, after expression of mRuby and mCherry in HeLa cells for 4 days, we observed punctate fluorescent labelling that resembled lysosomal localization, as previously described by Miyawaki et al . [12] This observation confirms our previous data for mCherry, although it should be mentioned here that in our previous work the punctate labelling was defined as ‘aggregates’ [6] . In contrast, we did not observe lysosomal localization of mKate2 and FusionRed after 4 days of expression under the same conditions ( Supplementary Fig. S5 ). To estimate relative protein toxicity at the whole organism level, Xenopus laevis embryos injected with plasmids expressing the actin and vimentin fusions of the tested fluorescent proteins were used as a laboratory animal model. In preliminary experiments, we observed various degrees of reduction of the average eye size, frequently accompanied by an unclosed optic fissure, in tadpoles expressing different fluorescent proteins (data not shown). The eye formation is a complex multistage process that depends on many mechanisms, any disturbance of which may result in an abnormal phenotype. Therefore, here we used eye development as a sensitive readout of possible abnormal course of embryogenesis caused by EGFP, FusionRed and mCherry expression ( Fig. 4a–h and Supplementary Tables S1–S3 ). In these experiments, actin and vimentin fusions of EGFP and FusionRed were only slightly more toxic than the uninjected controls, whereas expression of mCherry fusions led to notable decrease of the average eye size ( Fig. 4f ). Moreover, in many cases (80% of tadpoles with the reduced eye size), the reduced eye phenotype was accompanied by varying degree of an unclosed optic fissure, indicating an abnormal eye development ( Fig. 4g ). Together with the correlating toxicity data on the HeLa cells ( Fig. 4i ), superior performance in fusions ( Fig. 3 and Supplementary Fig. S4 ) and absence of abnormal lysosomal localization ( Supplementary Fig. S5 ), these results indicate that FusionRed is the least toxic of the tested red fluorescent proteins when expressed in living cells and organisms. This characteristic should improve the results of experiments that require long-term imaging of fused proteins of interest, including those in transgenic laboratory animals. The results described here should be also useful in future optimization of a number of TagRFP- and mKate-based proteins, including TagRFP-T [13] , mNeptune [9] , TagRFP657 (ref. 14 ), TagBFP [15] , LSS-mKates [16] , PATagRFP [17] , rsTagRFP [18] and KFP-HC [19] . Considering that all of these proteins are derivatives of mKate or TagRFP, and were not subjected to further engineering to improve monomeric character, they obviously do not share the purely monomeric (that is, at 10 mg ml −1 at HPLC) properties at this point. Thus, future derivatives could be developed using the results of this work to provide reliable performance for practical in vivo use. We believe that FusionRed will not only be useful by itself, but will serve a basis for development of new effective reporters for protein localization, multicolour imaging, FRET-based methods and as a core for novel red fluorescent biosensors. Labelling efficiency for FusionRed and mCherry HeLa CCL2 cells were cultured in Dulbecco’s modified Eagle’s medium (Invitrogen) supplemented with 12.5% fetal bovine serum (HyClone). Cells were then seeded onto square-shaped 18-mm coverslips inside 35-mm tissue culture dishes. Approximately 24 h after being seeded, cells were then transfected with 1 μg of DNA using Effectene (Qiagen) and maintained in a humidified 5% CO 2 incubator for at least 24 h before fixation. Cells were fixed with 3.7% paraformaldehyde and rinsed three times with glycine in phosphate-buffered saline to remove unreacted aldehydes. After fixation, coverslips were mounted in a polyvinyl alcohol medium and allowed to dry before imaging. Imaging was performed on a Nikon 80i upright microscope equipped with a X20 objective (numerical aperture = 0.75), a Semrock Texas Red filter set and a Hamamatsu Orca-ER camera. A single image of a randomly chosen viewfield filled with as many fluorescing cells as possible was acquired. Multiple viewfields were randomly imaged until an average of 150–200 properly expressing cells were imaged. Images were then inspected for the number of transfected cells and the number of properly expressing cells. The ratio of properly expressing cells versus the number of transfected cells was then used to calculate an average percentage of proper expression. Fluorescent proteins characterization in vitro Proteins fused to the N-terminal polyhistidine tag were expressed in Escherichia coli XL1 Blue strain (Invitrogen). The bacterial cultures were centrifuged and the cell pellets resuspended in 20 mM Tris–HCl, 100 mM NaCl, pH 7.5 buffer and lysed by sonication. The recombinant proteins were purified using TALON metal-affinity resin (Clontech) followed by a desalting step over gel filtration columns (Bio-Rad). Absorption spectra were recorded with a Beckman DU520 UV/VIS Spectrophotometer. A Varian Cary Eclipse Fluorescence Spectrophotometer was used for measuring excitation-emission spectra. All measurements were performed in buffer 100 mM NaCl, 20 mM Tris–HCl, pH 7.5. For molar extinction coefficient determination, we relied on measuring mature chromophore concentration. Proteins were alkali-denatured with an equal volume of 2 M NaOH and absorbance spectra were measured immediately. It is known that alkali-denatured DsRed-like chromophore converts to the GFP-like one [20] , with an extinction coefficient 44,000 M −1 cm −1 at 452 nm under these conditions. On the basis of the absorption of the native and alkali-denatured proteins, molar extinction coefficients for the native states were calculated. FusionRed is characterized by partial backbone cleavage before the Met of chromophore, analogous to asFP595 (asulCP, asCP) [21] , see Supplementary Figs S2,S3 . asFP595 wild-type protein contains 100% cleaved chromophore form and is characterized with molar extinction coefficient at 567 nm of 150,000 M −1 cm −1 (ref. 22 ). Absorbance of alkali-denatured asFP595 chromophore at 380 nm is 47% of asFP595 absorption at 567 nm at pH 7.5 and thus was determined as 70,000 M −1 cm −1 . Considering the relative input of peaks at 380 nm (extinction coefficient of this chromophore form = 70,000 M −1 cm −1 ) and 450 nm (extinction coefficient of this chromophore form = 44,000 M −1 cm −1 ) of FusionRed in alkaline conditions ( Supplementary Fig. S2 ), molar extinction coefficient of FusionRed at 580 nm was determined as 94,500 M −1 cm −1 . For determination of the quantum yield, the fluorescence of the mutant variants was directly compared with mCherry (quantum yield 0.22), and corrected to the area of the peak. pH titrations were performed by using a series of buffers in the range from 3 to 10. For each pH value, an aliquot of purified protein was diluted in an equal volume of the corresponding buffer solution and the fluorescence brightness was measured after 1 h incubation at room temperature. For accuracy, the actual pH was measured in each sample using a microelectrode (Sartorius). To measure the maturation rate, transformed E. coli cells (XL1 Blue strain) were grown overnight in LB supplemented with ampicillin and 2% D -glucose. Tubes were filled to the rim and sealed upon induction to restrict oxygen availability. The bacterial cultures were centrifuged and the cell pellets were resuspended in 20 mM Tris–HCl, 100 mM NaCl, pH 7.5 buffer and lysed by sonication. The recombinant proteins were purified using TALON metal-affinity resin (Clontech). Maturation was performed at 37 °C in 35 mM KCl, 2 mM MgCl 2 , 50 mM Tris pH 7.5, 1 mM DTT. A Varian Cary Eclipse Fluorescence Spectrophotometer was used for measuring maturation kinetics. High-performance liquid chromatography (HPLC) of the selected fluorescent proteins was performed on Varian 210 chromatograph. Gel filtration chromatography was performed using a Superdex 200 10/300 GL column (GE Bioscience), equilibrated with 40 mM Tris–HCl (pH 7.5), 150 mM NaCl buffer at a flow rate of 0.4 ml min −1 . Varian ProStar 335 flow spectrophotometer and Varian ProStar 363 flow fluorimeter were used for the detection. Apparent molecular masses were calculated by interpolating an elution volume versus log (molecular mass) calibration curve using ferritin (440 kDa), catalase (232 kDa), aldolase (158 kDa), bovine serum albumin (67 kDa), ovalbumin (43 kDa), chymotrypsinogen A (25 kDa), and ribonuclease A (13.7 kDa). Two hundred microlitre of each fluorescent protein at concentration 10 mg ml −1 were loaded. Microscopy All filters for fluorescence screening and imaging were purchased from Chroma Technology, Omega Filters or Semrock. HeLa epithelial (CCL-2, ATCC, Manassas, VA, USA) and grey fox lung fibroblast (CCL-168, ATCC) cells were grown in a 50:50 mixture of DMEM (Dulbecco’s modified Eagle’s medium) and Ham’s F12 with 12.5% Cosmic calf serum (Hyclone) and transfected with Effectene (Qiagen). Imaging was performed in Delta-T culture chambers (Bioptechs) under a humidified atmosphere of 5% CO 2 in air. Imaging in widefield mode was performed with a Nikon TE-2000 inverted microscope equipped with Omega QuantaMaxTM filters and a Photometrics Cascade II camera or an Olympus IX71 inverted microscope equipped with Semrock BrightLineTM filters and a Hamamatsu ImagEMTM camera. Laser-scanning confocal microscopy was conducted using a Nikon C1Si and an Olympus FV1000, both equipped with argon-ion (457 and 488 nm) and helium–neon or diode (543 and 561 nm, respectively) lasers and proprietary filter sets. Spinning disk confocal microscopy was performed on an Olympus DSUIX81 equipped with a Lumen 200 illuminator (Prior Scientific), a Hamamatsu 9100-13 EMCCD camera, Semrock filters and ten position filter wheels driven by a Lambda 10-3 controller (Sutter). In some cases, cell cultures expressing fluorescent protein fusions were fixed after imaging in 2% (w/v) paraformaldehyde (electron microscopy sciences) and washed several times in phosphate-buffered saline containing 0.05 M glycine before mounting with a poly (vinyl alcohol)-based medium. Morphological features in all fusion constructs were confirmed by imaging fixed-cell preparations on coverslips using a Nikon 80i upright microscope and Semrock Texas Red filter set (4040B) coupled to a Hamamatsu Orca ER or a Photometrics CoolSNAPTM HQ2 camera. Estimation of cytotoxicity Cell analysis was performed using a Cytomics FC 500 (Beckman Coulter) flow cytometer. Data were analyzed using the program Cytomics RXP Analysis (Beckman Coulter). Toxicity in Xenopus laevis embryos Xenopus laevis embryos were staged according to [23] . Plasmids were purified by Qiagen columns and phenol/chlorophorm extraction followed by ethanol precipitation. Plasmid DNA (15 pg per blastomer) was injected at eight-cells stage into animal regions of two dorsal blastomeres by Eppendorf FemtoJet microinjector. In sum, more than 90 embryos for each type of plasmids were injected in three independent series of experiments. To standardize injections made by different micropipettes, we used the following procedure. Plasmids were diluted to 3.6 μg μl −1 and pressure in the microinjector was adjusted so that each injection pulse squeezed from the micropipette tip a drop with the diameter of 200 μm (the value corresponding to five small divisions of the eyepiece scale at the magnification used for injections). The selected diameter of the drop corresponds to the volume of about 4.2 nl, which in turn corresponds to 15 pg of a plasmid. Calibration procedure was performed for each micropipette before the beginning of injections. Thus, uniform injection conditions for all micropipettes were provided regardless of possible variations in their individual characteristics. Moreover, in the process of injections, we periodically controlled the uniformity of the procedure by taking out the micropipette from the Ficoll solution (4% Ficoll, 0.1 MMR) after injections into each four to five embryos and measuring the diameter of the drop squeezed from its tip by the eyepiece scale. If size of the drop appeared to be larger or smaller than five divisions of the eyepiece scale, we adjusted it to this value by adjusting pressure. The uniformity of injections was additionally controlled by discarding embryos that demonstrated at the tailbud stage too high or too weak signal of the in vivo tracer, which was premixed with injected plasmids: fluorescein-lysine-dextran (Invitrogen, 40 kDa, final concentration 3 mg ml −1 ) in case of plasmids expressing red fluorescent proteins, and rhodamine-lysine-dextran (Invitrogen, 10 kDa, final concentration 10 mg ml −1 ) in case of actin-EGFP plasmid. All experiments were repeated in three independent series (in three different days, see Supplementary Tables S1–S3 ). Embryos were incubated in 0.1 MMR until stage 41, photographed by M205 Leica fluorescent stereomicroscope with TexasRed and GFP filter sets and images were analyzed by LAS software. See Supplementary Methods for further details. How to cite this article : Shemiakina I.I. et al . A monomeric red fluorescent protein with low cytotoxicity. Nat. Commun. 3:1204 doi: 10.1038/ncomms2208 (2012).